Morphology of seahorse head hydrodynamically aids in capture of evasive prey Syngnathid fish (seahorses, pipefish and sea dragons) are slow swimmers yet capture evasive prey (copepods) using a technique known as the ‘pivot’ feeding, which involves rapid movement to overcome prey escape capabilities. However, this feeding mode functions only at short range and requires approaching very closely to hydrodynamically sensitive prey without triggering an escape. Here we investigate the role of head morphology on prey capture using holographic and particle image velocimetry (PIV). We show that head morphology functions to create a reduced fluid deformation zone, minimizing hydrodynamic disturbance where feeding strikes occur (above the end of the snout), and permits syngnathid fish to approach highly sensitive copepod prey ( Acartia tonsa ) undetected. The results explain how these animals can successfully employ short range ‘pivot’ feeding effectively on evasive prey. The need to approach prey with stealth may have selected for a head shape that produces lower deformation rates than other fish. Syngnathid fish (e.g., seahorse, pipefish and sea dragons) are slow swimmers, yet capture evasive prey [1] , [2] with high success [3] . Planktonic copepods, a common food source of syngnathid fish [4] , possess powerful and effective escape responses to the approach of predators [5] , [6] . Mechanoreception of hydrodynamic disturbances, flow shear (strain), is considered most important for the remote detection and discrimination of predators [7] , [8] , [9] , [10] . Copepods can respond to these hydrodynamic signals within 2–4 ms [5] , [11] , [12] and achieve escape speeds over 500 body lengths per second [5] , [13] . Successful capture of evasive prey in syngnathids is attributed to a two-phase prey-capture mechanism that is commonly referred to as pivot feeding [14] , [15] , [16] , [17] . This consists of rapid upward rotation of the head in combination with suction to draw the prey into the seahorse’s mouth. Because suction only works within a relatively short distance of the mouth [18] , syngnathid fish must bring the mouth close to the prey quickly by rotating the head which is critical to prey capture. To accomplish this, syngnathid fishes (seahorses, pipefish and sea dragons) are equipped with large tendons that has been proposed to store and release elastic energy to accelerate the head rapidly towards the prey [16] . The S-shaped body of the seahorse also aids in this rapid upward thrust of the mouth [19] . However, this mechanism only works at close range [18] , [20] , and thus the seahorse must approach very close to the prey in order for a strike to occur. Thus, before a strike can be successful, syngnathid fish must first approach without hydrodynamically alerting evasive prey. This feeding method is different from many planktivorous fish predators that often use highly protrusive jaws [21] , [22] , [23] and/or rapid lunges [24] . The dwarf seahorse, Hippocampus zosterae, similar to other syngnathidae, dwell within seagrass beds or sheltered habitats, where water movement is dampened [25] . Copepod prey are sensitive to low fluid deformations, which is defined as the rate of change in strain (deformation) of a material, , where is the fluid velocity and is the spatial gradient. In water (incompressible fluid) this is the rate at which it is being deformed by progressive shearing (shear rate). Amid low ambient shear, the prey (copepods), with sensitive mechanoreceptors capable of detecting deformation rates of ≈0.5 s −1 (refs 12 , 26 , 27 ) can sense and respond to hydrodynamic disturbances at greater distances relative to turbulent environments [28] . In such an environment, a predator must approach prey with stealth. This is exemplified by planktivorous reef fish (blennies) in which success rates of copepod capture drop from 56% in turbulent conditions (natural environment) to 21% in calm conditions [24] . In this study, we test the hypothesis that head morphology of the dwarf seahorse is not only adapted for a quick strike but also provides a hydrodynamic advantage when approaching evasive prey. Using the high speed digital holographic techniques [29] with live animals, we measure 3D movements of H. zosterae and Acartia tonsa while simultaneously measuring fluid motion at the plane of interest. This provides qualitative evidence of a zone located above the snout within the strike zone, where flow motion is lower than surroundings. Using Particle Image Velocimetry (PIV) and preserved fish in flume experiments, we present quantitative data demonstrating head morphology of the dwarf seahorse, combined with posture serves to minimize hydrodynamic disturbance during approaches and to position prey undetected within the zone where rapid pivot feeding is effective. We also test a phylogenetic relative lacking an elongated snout, the stickleback ( Gasterosteus aculeatus ), and neither morphology nor posture generates a hydrodynamically quiet zone where strikes occur. Interactions with live prey Eighty-four percent of approaches by H. zosterae resulted in the copepod ( A. tonsa ) becoming successfully positioned within strike range (≈1 mm) without triggering an escape response. Successful approaches occur at speeds of 8.4±6.1 mm s −1 which is significantly lower ( P =0.009 t -test, n =25) than that of unsuccessful predation attempts at 14.1±8.4 mm s −1 ( Fig. 1a ). Once within range, pivot feeding resulted in capture success of 94% (attempts that resulted in both successful approach and strike=79%). High speed holographic recordings (2,000 Hz) revealed the seahorse’s mouth covered the distance to the copepod in <1 ms ( Figs 2a and 3a,b ). 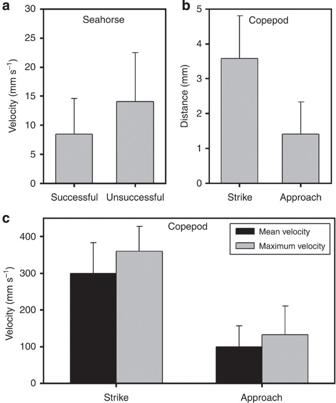Figure 1: Kinematic results of feeding attempts byH. zosteraeonA. tonsa. Error bars represent s.d. andn=15 for each case. (a) Approach velocities of the seahorse during successful and unsuccessful feeding attempts. (b) Copepod escape distance in response to an approach and escape distance by adjacent copepods to a feeding strike. (c) Escape velocities for copepods responding to an approach and adjacent copepods that responded to the feeding strike. Figure 1: Kinematic results of feeding attempts by H. zosterae on A. tonsa . Error bars represent s.d. and n =15 for each case. ( a ) Approach velocities of the seahorse during successful and unsuccessful feeding attempts. ( b ) Copepod escape distance in response to an approach and escape distance by adjacent copepods to a feeding strike. ( c ) Escape velocities for copepods responding to an approach and adjacent copepods that responded to the feeding strike. 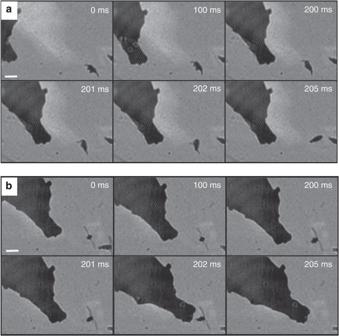Figure 2: Reconstructed high speed holographic video frame sequence ofH. zosteraefeeding onA. tonsa. Scale bar=1 mm. (a) Unsuccessful feeding attempt where the approach of the seahorse was detected by the copepod. (b) Successful feeding attempt resulting in a rapid strike and ingestion of the copepod. Full size image Figure 2: Reconstructed high speed holographic video frame sequence of H. zosterae feeding on A. tonsa . Scale bar=1 mm. ( a ) Unsuccessful feeding attempt where the approach of the seahorse was detected by the copepod. ( b ) Successful feeding attempt resulting in a rapid strike and ingestion of the copepod. 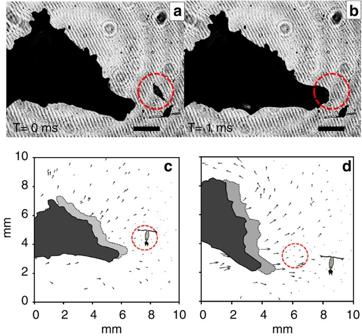Figure 3: Interactions of live seahorse with copepods recorded with high speed digital holography. Scale bar=1 mm. (a) Holographic in-focus image ofH. zosteraethat has successfully approachedA. tonsaand positioned the copepod within the strike zone. Scale: 1 mm. The strike (b) occurs via rapid pivot feeding and successfully captures the copepod. The strike region (red) is enclosed by a dashed line and particle tracks are highlighted as solid lines: (c) a successful approach showing a rendered depiction of the actual diatom streak-lines (black) from superimposed holographic images. Particle velocity did not exceed 0.8 mm s−1at any point within the strike zone. (d) An unsuccessful approach with greater velocity within the strike zone (4.1±1.5 mm s−1) and alerted the copepod to the presence of a potential predator. Full size image Figure 3: Interactions of live seahorse with copepods recorded with high speed digital holography. Scale bar=1 mm. ( a ) Holographic in-focus image of H. zosterae that has successfully approached A. tonsa and positioned the copepod within the strike zone. Scale: 1 mm. The strike ( b ) occurs via rapid pivot feeding and successfully captures the copepod. The strike region (red) is enclosed by a dashed line and particle tracks are highlighted as solid lines: ( c ) a successful approach showing a rendered depiction of the actual diatom streak-lines (black) from superimposed holographic images. Particle velocity did not exceed 0.8 mm s −1 at any point within the strike zone. ( d ) An unsuccessful approach with greater velocity within the strike zone (4.1±1.5 mm s −1 ) and alerted the copepod to the presence of a potential predator. Full size image Unsuccessful feeding strikes occurred at a significantly ( P =0.01, t -test, n =15) greater distance (1.2 mm s.d. 0.18) than did successful strikes (0.89 mm s.d. 0.22). No strikes on A. tonsa were observed at distances exceeding 1.4 mm. Of the copepods that responded to the approach of the seahorse (e.g. Fig. 2a ), the escape jumps often resulted in only a single metachronal swimming stroke of the thoracic pereiopods and these escapes exhibited mean velocities of 99 mm s −1 (s.d. 57) and maximum velocities of 132 mm s −1 (s.d. 79) ( Fig. 1c ). This is significantly lower ( P <0.001, t -test, n =20) than the response of copepods adjacent to the seahorse, which responded to the rapid feeding strike with multiple swimming strokes and escaped at a mean velocity of 300 mm s −1 (s.d. 82) and maximum velocity of 360 mm s −1 (s.d. 68). Response distance was also significantly higher ( P =0.01, t -test, n =20) for reactions of copepods to strikes compared with copepods that react to approaches ( Fig. 1b ). The maximum measured reaction distance to an approach from H. zosterae was 1.6 mm (mean 1.5 mm, s.d. 0.1), whereas responses to a strike occurred up to 4.4 mm away from the seahorse (mean 2.5 mm, s.d. 1.3). Fluid motion around live fish To obtain a general sense of fluid motion produced during predatory approaches of live H. zosterae towards copepods ( A. tonsa ), we compared fluid velocity within and directly adjacent to the strike region, at the z plane of the prey. Reduced fluid motion within the strike region was observed in both successful and failed approaches ( Fig. 3c,d ). Results from 15 predatory approaches by H. zosterae (six individuals) show that within the empirically defined boundaries of the strike region, fluid velocities did not exceed 0.8 mm s −1 , whereas adjacent regions exhibited velocities of 4.1 mm s −1 (s.d. 1.5). The result is that fluid motion within the strike region is significantly lower ( P <0.001, t -test). The orientation of the seahorse’s head posture relative to the copepod was consistent during predatory approaches. The angle formed from the top of the head to the tip of the snout to the centre of the copepod was 124.3° (s.d. 4.1, n =21). This orientation remained consistent throughout the approach as rotation of the head during this period was ≤3.3°. Flume study Results from the PIV flume experiments with preserved specimens of H. zosterae confirmed the presence of a low deformation rate zone, and that the greatest hydrodynamic disturbance occurs near the top of the head and from the edge of the snout ( Fig. 4 ). The tested flow velocities, representing the range of observed approach speeds, reveal that overall, fluid deformation rates remain low in the strike region relative to surrounding areas, but increase with flow speed ( Fig. 4 ). At a flow velocity representing unsuccessful approaches on A. tonsa (20 mm s −1 ), influence from the head extends a greater distance and deformation rates ≥0.5 s −1 can be found in the majority of the strike region. At 10 mm s −1 , deformation rates ≥0.5 s −1 occur in only part of the strike region ( Fig. 4b ), whereas virtually no region of ≥0.5 s −1 exists in the strike region at 4 mm s −1 ( Fig. 4a ). 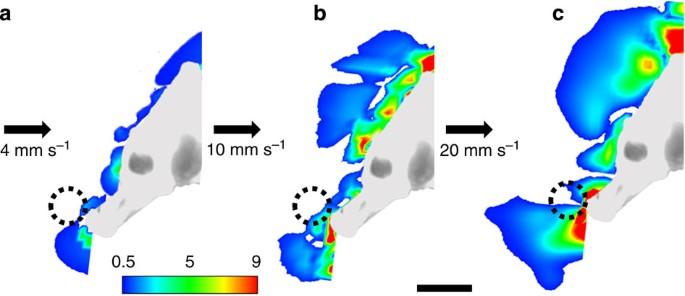Figure 4: Time-averaged results of deformation rates ≥0.5 s−1created by an approaching seahorse at different speeds. (a) 4 mm s−1(b) 10 mm s−1(c) 20 mm s−1. Here threshold for detection byA. tonsa(≥0.5 s−1) extends further from the head with flow speed but the strike zone (black circle) maintains low deformation rates relative to other areas around the head. Arrows indicate direction of water motion. Scale bar=2 mm andn=5. Figure 4: Time-averaged results of deformation rates ≥0.5 s −1 created by an approaching seahorse at different speeds. ( a ) 4 mm s −1 ( b ) 10 mm s −1 ( c ) 20 mm s −1 . Here threshold for detection by A. tonsa (≥0.5 s −1 ) extends further from the head with flow speed but the strike zone (black circle) maintains low deformation rates relative to other areas around the head. Arrows indicate direction of water motion. Scale bar=2 mm and n =5. Full size image The effect of posture was also measured at a commonly observed approach speed (9 mm s −1 ). The head was positioned at various angles representing non-syngnathid posture, natural seahorse posture and downward facing posture. 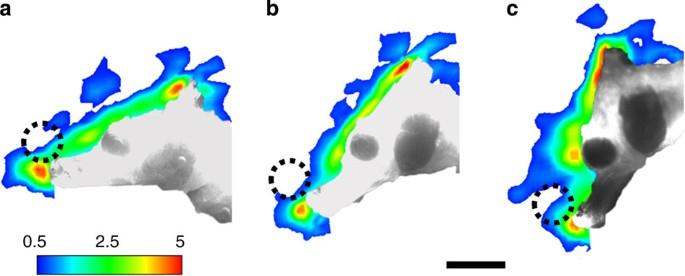Figure 5: Time-averaged results of deformation rates ≥0.5 s−1created by an approaching seahorse at the speed of ~10 mm s−1. Scale bar=2 mm,n=5. (a) Head angled straight to simulate the approach posture of other planktivorous species. (b) Natural posture when approaching prey. (c) Head angled downwards. The strike zone is indicated by a black circle. Figure 5 shows that fluid deformation is consistently lower in the strike region relative to measurements at the leading edge of the snout and head (in front of the eye) irrespective of head angle ( Fig. 5 ). However, posture also has a role because fluid deformation rates are lowest within the strike region of the naturally observed posture. Fluid deformation and the effect of posture were also measured for the three-spined stickleback G. aculeatus , taxonomic relative without an elongated snout. 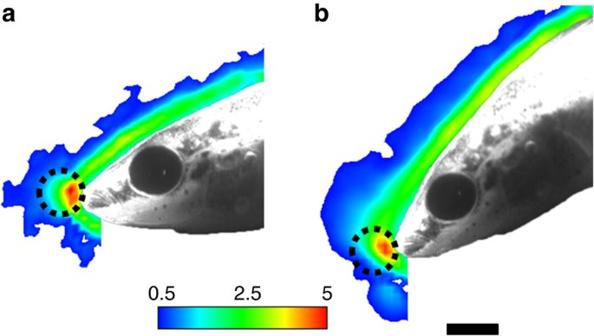Figure 6: Time-averaged results of deformation rates ≥0.5 s−1created by an approaching three-spined stickleback at a speed of ~10 mm s−1. Scale bar=2 mm,n=5. (a) Natural posture when approaching prey. (b) Head angled downwards to represent the posture of a seahorse approaching prey. The strike range of the seahorse is indicated by a black circle. Figure 6 shows the presence of relatively uniform bow wave produced by this morphology, with greatest deformation rates occuring directly in front of the mouth. The effect of posture does not greatly influence deformation rates at the strike range observed in seahorses ( Fig. 6b ). Figure 5: Time-averaged results of deformation rates ≥0.5 s −1 created by an approaching seahorse at the speed of ~10 mm s −1 . Scale bar=2 mm, n =5. ( a ) Head angled straight to simulate the approach posture of other planktivorous species. ( b ) Natural posture when approaching prey. ( c ) Head angled downwards. The strike zone is indicated by a black circle. Full size image Figure 6: Time-averaged results of deformation rates ≥0.5 s −1 created by an approaching three-spined stickleback at a speed of ~10 mm s −1 . Scale bar=2 mm, n =5. ( a ) Natural posture when approaching prey. ( b ) Head angled downwards to represent the posture of a seahorse approaching prey. The strike range of the seahorse is indicated by a black circle. Full size image We find that once H. zosterae is within range (≈1 mm) of a copepod, capture success is 94%. The high rate of capture is due to the unique method of strike known as ‘pivot’ feeding [14] , [16] , [17] , [19] , [30] , which relies on a four-bar linkage of cranial components [20] , [31] , [32] and large tendons of the epaxial muscles, which are hypothesized to store and release elastic energy to accelerate the head [17] , [33] . This is supported by our data that show that copepods within the strike region have little chance at escape as pivot feeding covers the distance to the copepod in <1 ms ( Fig. 3a,b ), faster than the 2–4 ms response latency of the copepod [5] . However, although the use of pivot feeding to explain the adaptive significance of head morphology in sygnathid fish [19] is important, one cannot ignore the fact that without the ability to approach evasive prey undetected, short range pivot feeding becomes ineffective. The dwarf seahorse, H. zosterae , is found within seagrass beds [34] that dampen water motion and reduces turbulence [25] , [35] . This will allow copepods to respond at greater distances [28] , and it is reasonable to expect that sensitivity to hydrodynamic disturbances is close to their detection limit. In addition, these fish must approach a copepod to within ≈1 mm in order to strike ( Fig. 3a ). This creates a challenging situation for a predator. We find H. zosterae successfully positions A. tonsa within the strike region 84% of the time without generating an escape response. The use of live animals and holographic techniques provides qualitative evidence of a reduced fluid disturbance in the strike region relative to surrounding areas of equivalent distance to the head ( Fig. 3c,d ). This creates a weaker hydrodynamic signal (deformation rate) in the strike region available for detection by prey and likely decreases the probability of copepods sensing an approach. It is important to consider, however, that this area of the reduced fluid motion in the strike zone is flanked above and below by areas of elevated fluid disturbance so positioning of prey during an approach is important as the fish must orient appropriately to avoid detection. To more robustly test the assertion that head morphology alone can provide hydrodynamic stealth, preserved specimens were used in flume experiments with planer (2D) PIV. We observed elevated deformations rates in the strike zone as approaching speed increases ( Fig. 4a–c ), thereby increasing the probability of alerting prey and thus diminishing capture success. However, even at the greatest simulated approach speed, 20 mm s −1 , the head morphology maintains comparatively low fluid deformation rates within the strike zone. Copepods are known to respond with submaximal velocities to relatively weak hydrodynamic signals [36] and this could explain why copepods that sensed the approach of the seahorse and responded with an escape jump, performed only ≤2 swimming strokes and mean escape velocities of only 99 mm s −1 (s.d. 57). These velocities were significantly weaker than adjacent copepods responding to a feeding strike (stronger hydrodynamic signal) and exhibited mean velocities of 300 mm s −1 (s.d. 82) ( Fig. 1c ). Thus, even if the seahorse approach is detected, the copepod is unlikely to leave the predator’s perceptive field resulting in multiple attacks ( Supplementary Movie 1 ). Figure 4a–c show regions where deformation rate exceeds the detection sensitivity of copepod A. tonsa , which is one of the most sensitive copepod species to hydrodynamic disturbance and responds to low threshold deformation rates [12] , [26] , [27] . It is important to consider that, although the threshold of 0.5 s −1 may elicit an escape response by A. tonsa , other species require greater deformation rates to escape [12] , [27] . Thus, success on a wide range of prey is possible, even at the highest observed approach speeds, because head morphology maintains shear stress distribution within the strike zone even at higher detection thresholds. We find that H. zosterae consistently positions the head relative to prey at a specific orientation. Results from varying the head posture in flume studies demonstrate that fluid deformation is consistently lower in the strike region relative to measurements at the leading edge of the snout and head (in front of the eye) irrespective of the head angle ( Fig. 5 ). At the flow speed tested (~9 mm s −1 ) this allows at least part of the strike region in all cases to exhibit low disturbance and suggests that morphology has a role in reducing fluid disturbance at a wide range of postures. However, posture also has an important role. At an approach angle of most mid-water planktivores ( Fig. 5a ), fluid strain is elevated in the strike zone compared with the observed approach angle ( Fig. 5b ). A similar change occurs when angle of the head is too steep ( Fig. 5c ). Therefore, although morphology alone is capable of producing a ‘quiet zone’ at a variety of approach angles, posture can aid in optimizing this effect. How do the results on seahorse head morphology compare with other fish morphologies? A study comparing seahorse morphology to that of a salmon found that the seahorse model induced the lowest number of prey escape responses [37] . When both models were presented to mysids ( Paramesopodopsis rufa ) at the same speed, the model based on salmon morphology elicited escape responses by prey, whereas the seahorse did not. A study on Bluegill ( Lepomis macrochirus ), which exhibits common head morphology of planktivorous fish, found that they approached copepods at 11 mm s −1 (nearly identical to H. zosterae in the current study), yet the minimum deformation rates measured at 1 to 2 mm from the head was ≥5 s −1 , and deformation rates below copepod detection (≤0.5 s −1 ) do not occur until >5 mm in front of the head [23] . The bluegill can still effectively capture copepods because strikes occur when prey is 8.13 mm (s.e. 0.54) away from the mouth, where fluid deformation is still low and prey have not received sufficient hydrodynamic signals for escape. The use of protrusive jaws allows bluegill to cover this distance. For H. zosterae , generating such hydrodynamic disturbance close to the head would result in many copepods detecting an approach before a strike can be initiated as strike distance of this species is <1.4 mm. Therefore, the seahorse morphology is adapted to further minimize hydrodynamic disturbances and at velocities near 10 mm s −1 , much of the strike region (zone of minimum deformation), located 1 to 2 mm from the mouth exhibits deformation rates ≤0.5 s −1 . A study investigating copepod responses to fluid disturbance by another ancestral zooplanktivorous fish morphology (juvenile salmon) quantified deformation rates around the head and found that the strongest fluid strain occurs directly in front of the mouth, where strikes occur [38] . Although previous studies suggest a fundamental difference in the hydrodynamic profiles generated by the seahorse morphology versus other fish that feed on copepods, it is useful to compare deformation profiles with a close phylogenetic relative without an elongated snout. Results from the current study show that the three-spined stickleback ( G. aculeatus ) produces comparatively high fluid deformation rates in the region where strikes occur ( Fig. 6a ). In addition, if a stickleback were to approach prey with the posture/angle of a seahorse, a large bow wave is still formed at the leading edge, and if the strike range is similar to a seahorse, the entire strike zone exceeds the strain threshold for escape responses by evasive copepods ( Fig. 6b ). Therefore, the morphology of the seahorse head allows for the creation of a hydrodynamically quiet zone that cannot be achieved through changes in posture with morphologies of other suction feeding predators of copepods. The hydrodynamic advantage of the seahorse morphology likely arises from the fact that the mouth is positioned at the end of a thin structure, at some distance away from the head. This thin, elongated snout will allow fluid to pass more easily (thus lower deformation develops here) than when the mouth is directly attached to a more blunt head. The result is a zone of reduced hydrodynamic disturbance between the leading edge of the mouth and the head. An upturned mouth and a pivot feeding strike mechanism that rotates the head rapidly upwards allow the seahorse to take maximum advantage of this hydrodynamically ‘quiet’ region. In other species that feed on evasive copepods, a large bow wave is observed directly in front of the mouth where strikes occur and highest fluid deformations also occur here ( Fig. 6 ). Thus, neither morphology nor posture in these taxa acts to reduce hydrodynamic disturbance in the strike zone. However, we know these fish can still successfully capture evasive copepods. Likely, the use of highly protrusive jaws during the strike phase allows these species to cover greater distances than seahorses [23] , and hence higher deformation rates near the mouth may become less of a problem. It is also possible that these species employ a mechanism known as the ‘compensatory suction’ that has been proposed in turtles [39] . If also present in fish, it may also act to help offset the greater disturbance generated by a comparatively blunt morphology. Instead of highly protrusive jaws or compensatory suction, syngnathid fish successfully use morphology to facilitate successful strikes via pivot feeding. One possibility for why pivot feeding in syngnathid fish evolved from the ancestral protrusion method is that the strike time of pivot feeding (≤1 ms in current study) is faster than protrusive feeding that takes ≥10 ms [40] . This allows pivot feeders (syngnathids) to strike faster than the response latency of their prey. Thus, we find that once the prey is within strike range capture success is nearly 100%. However, this mechanism works only at short ranges so getting close to hydrodynamically sensitive, evasive prey without triggering an escape response becomes imperative. This is most critical in low turbulence environments such as seagrass beds, where hydrodynamically sensitive prey can more easily detect an approaching predator. Ancestral morphologies and feeding methods can still be effective here, but may function most efficiently in more turbulent environments. Both holographic and PIV measurements provide evidence that head morphology of H. zosterae produces low deformation rates within the strike zone to facilitate rapid ‘pivot’ feeding. The unique morphology of syngnathid fish provides an advantage to a slow moving, cryptic predator and may explain the adaptive significance for the unique head structure found within this group of organisms. This morphology may also have implications in bio-inspired designs of microstructures for microfluidics applications and flow assisted cell manipulations, where low-shear zones are required. Experimental setup Copepods were collected from coastal waters of the Gulf of Mexico (27°50′19′′N 97°3′8′′W) using a 0.5 m diameter and 150 μm mesh plankton net. Adult A. tonsa copepods (prosome length 0.8–1.1 mm) with intact antennae were sorted from other zooplankton species. Specimens of the dwarf seahorse, H. zosterae , (standard length≈2.5 cm) were acquired from the Fisheries and Mariculture Laboratory at the University of Texas at Austin Marine Science Institute. Only preserved specimens of the three-spined stickleback ( G. aculeatus ) were used in this study and were obtained from the Marine Biological Laboratory (Woods Hole, USA). Experiments with live animals were conducted in a small glass aquarium (inside dimensions 4 × 4 × 4 cm) constructed of low-iron glass for optimal image quality. Filtered seawater used in the experiments was seeded with cultured, neutrally buoyant, live diatoms ( Thalassiosira sp., diameter ≈15 μm) to a density of ~100 cells per ml. The diatoms serve two functions: to act as a flow tracer and to also provide a natural food source for the copepods to elicit more natural behaviour under experimental conditions. Experimental protocols were approved by the Institutional Animal Care and Use Committee at the University of Texas at Austin. The seahorse was provided a cylindrical plastic rod (1.5 mm diameter) attached to a base in the middle of the aquarium to grasp with its prehensile tail when feeding. Experiments were performed in a darkened room and ambient white lighting was supplied by a Fisher Scientific fibre optic illuminator ( ca . 150 μM m −2 s −1 ) in a vertical beam from above. This provided illumination for the visually hunting fish and because the light attracts copepods, the beam was used to orient the fish’s feeding attempts perpendicular to the field of view of the video camera in order to obtain flow measurements around the fish’s head. Holography Digital in-line holography ( Fig. 7a ) was used to provide flow measurements around the head of the live seahorse H. zosterae and track the 3D trajectory of prey ( A. tonsa ). This method is described in detail in [29] and summarized below. 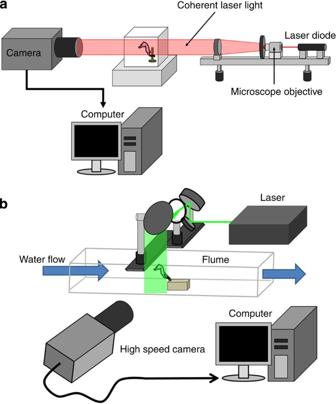Figure 7: Experimental set ups. (a) In-line holographic system used to generate a collimating, coherent beam and to record the interference pattern to produce 3D holographic images. (b) PIV. A vertical laser sheet (532 nm) is projected downwards through the flume and was centred over the sagittal plane of the seahorse. Note: diagrammatic (not to scale). Figure 7: Experimental set ups. ( a ) In-line holographic system used to generate a collimating, coherent beam and to record the interference pattern to produce 3D holographic images. ( b ) PIV. A vertical laser sheet (532 nm) is projected downwards through the flume and was centred over the sagittal plane of the seahorse. Note: diagrammatic (not to scale). Full size image Both 2D and 3D standard video techniques are limited to relatively narrow focal planes, and therefore objects moving freely in water will be in-focus for only a short period. The holographic technique provides a means to capture detailed sequences of objects in 3D with a single camera, no matter the object location within the field of view. In the context of this study, digital holography provides the ability to obtain flow field information around the head of a feeding seahorse no matter its depth of field location and track locations of copepods during responses to the seahorse. Although the particles can be tracked in any plane, we used only instances where the seahorse fed perpendicular to the field of view because a single camera is used and therefore other orientations of the fish can visibly block the region of interest. Digital holography is based on a two-step process (hologram formation and numerical reconstruction). First, an in-line hologram was produced by back-illuminating a sample volume with a collimated, coherent light and recording the resulting diffraction pattern produced by objects in the field of view, on a CCD array within a high speed video camera. Coherent light is first focused through a pinhole to remove aberrations that may be present in the light source. This light then expanded and passed through a columnating lens to produce the constant diameter beam. A diffraction pattern is generated as a result of interference between the illuminating beam and light scattered from the objects. Coherence of the light source is important in order to enhance the visibility (or contrast) of the interference pattern, which conveys information on the shape and location of an object in space and collimating the expanded beam enables recording of the diffraction patterns at a constant magnification [29] . The recorded image contains the result of interference between the undisturbed part of the illuminating beam and the light scattered from objects in the sample volume. This contains all the information needed for reconstructing the location and shape of particles over the entire sample volume. The expanded beam of 2.5 cm diameter illuminated a 20 ml sample volume. A 0.5 mW (660 nm) laser diode was used because most marine organisms show low sensitivity to the red spectrum [41] , thereby minimizing changes in behaviour. The interference patterns (holograms) generated by the laser were recorded on a Photron SA3 high speed camera with a 1,024 × 1,024 pixel CCD sensor using a Nikon Nikkor 105 mm at 2,000 frames per second at a magnification of × 1. The holograms were reconstructed numerically using in-house developed software based on the Fresnel-Huygens transformation [29] , [42] . Characteristics of seahorse, prey and diatoms, positions, in-focus images and shapes were determined using a post-processing algorithm [43] . To visualize the flow, in-focus images at any given time were reconstructed at the spacing of 20 μm over a thickness of 2 mm centred at the plane of snout and coincidentally that of the copepod. These images were superimposed to produce a combined image showing all particle images located within a sample volume of 15 × 15 × 2 mm. The flow vectors shown by streak-lines of tracer particles at the in-focus plane of seahorse snout is obtained by superimposing reconstructed images over the final 100 frames (50 ms) during feeding approaches on the copepod, A. tonsa . Feeding attempts by the seahorse were monitored for success (copepod consumed) or failure (copepod escaped), although simultaneously the corresponding biogenic flow fields were recorded. Approach speeds were measured and statistical analysis was performed using Sigmaplot v11. Approach speed data were log transformed and checked for normality (Shapiro–Wilk test). A student’s t -test with alpha value 0.05 was used to compare approach speeds, copepod reaction distance and swimming velocity and fluid motion of successful and failed predation attempts. The strike region was empirically defined by measuring the observed strike distances of H. zosterae from the current study using ImageJ (v 1.45) software, and ranged from 0.5 to 1.4 mm. For comparisons of flow velocities of around live seahorses, we assume a circular strike region of 0.9 mm in diameter beginning at a distance of 0.5 mm from the head. Mean velocity within the region was obtained by averaging all vectors within the circular boundary. An identical circular region (0.9 mm diameter) was superimposed using the ImageJ directly adjacent to the strike region (also beginning 0.5 mm from the head). Flow vectors within this region were compared with the strike region using the Student’s t -test. Particle image velocimetry Systematic flow and morphology studies were conducted using PIV and a constant pressure-head, low-speed laminar flume ( Fig. 7b ). Five preserved specimens each of H. zosterae and G. aculeatus (≈3 cm TL) were mounted from a base so as to allow fine control over the orientation of the head relative to the flow. The head was such that the posture was similar to that species’ natural predatory approach and then also at several postures that deviated from this. Water was seeded with hollow, silver-coated glass beads (15 μm). An in-housed developed PIV system including a dual-head ND:YAG ( λ =532 nm) PIV laser (LithoNano), a 2Kx2K CCD camera (Imperex 4M15L) at 7 frame pairs per sec and beam shaping optics was used. The delay between two exposures was 20 ms. Instantaneous velocity maps were analysed by in-house developed PIV software (mCorePIV). Three flow conditions representing the range of approaching speed were selected. Each measurement condition was time averaged and consists of over 5,000 instantaneous PIV realizations recorded over a period of ~12 min that ensure robust measurements and that features in the deformation rate profiles are depicted accurately. Mean deformation rates created by the morphology of the seahorse head was estimated from the mean velocity field as the following: where U is the horizontal ( x ) velocity components and V the vertical ( y ) component. How to cite this article: Gemmell, B. J. et al. Morphology of seahorse head hydrodynamically aids in capture of evasive prey. Nat. Commun. 4:2840 doi: 10.1038/ncomms3840 (2013).